Visualization and genetic modification of resident brain microglia using lentiviral vectors regulated by microRNA-9 Functional studies of resident microglia require molecular tools for their genetic manipulation. Here we show that microRNA-9-regulated lentiviral vectors can be used for the targeted genetic modification of resident microglia in the rodent brain. Using transgenic reporter mice, we demonstrate that murine microglia lack microRNA-9 activity, whereas most other cells in the brain express microRNA-9. Injection of microRNA-9-regulated vectors into the adult rat brain induces transgene expression specifically in cells with morphological features typical of ramified microglia. The majority of transgene-expressing cells colabels with the microglia marker Iba1. We use this approach to visualize and isolate activated resident microglia without affecting circulating and infiltrating monocytes or macrophages in an excitotoxic lesion model in rat striatum. The microRNA-9-regulated vectors described here are a straightforward and powerful tool that facilitates functional studies of resident microglia. Microglia are a resident population of immune cells in the brain. In the adult brain, microglia are heterogeneously distributed throughout the central nervous system (CNS). This cell type constitutes between 5 and 12% cells in the rodent brain, depending on the brain region [1] . The microglia population has classically been associated with canonical CNS responses against pathogens and brain injuries [2] . However, recent studies have indicated that microglia have a more complex role in maintaining CNS homoeostasis than what was initially believed. For example, microglia have been demonstrated to influence neurogenesis and synapse formation [3] , [4] . Moreover, microglia can be primary agents of several diseases within the CNS, including Rett syndrome, for which recent studies have shown that microglia can drive disease phenotype in animal models [5] . Resident brain microglia originate from myeloid progenitors born during early development [6] . In addition, infiltrating monocyte-derived macrophages can enter the brain following insults or in disease, and recent studies suggest that these two cell populations have distinct roles in the brain [7] . The myeloid origin of microglia distinguishes them from other glial cell types such astrocytes and oligodendrocytes that have a neuroecteodermal origin [6] . The exact role of microglia in the healthy and diseased brain remains largely elusive, as it has been difficult to genetically modify the resident microglia population in a cell-type-specific manner [8] . The use of transgenic mice carrying tissue-specific promoters, bacterial artificial chromosome transgenes or knock-in cassettes to target genetic modifications to resident microglia, result in additional targeting of monocyte/macrophage populations throughout the body. This approach therefore does not allow a separation of function between these monocyte-derived macrophages and resident brain microglia. An alternative to transgenic mice could be brain injections of viral vectors, such as lentiviral vectors or adeno-associated viral vectors, to specifically target microglia [9] . Using either a cell-specific promoter or a capsid with tropism for microglial cells would allow for cell-specific genetic manipulation of resident microglia. However, such efforts have been largely unsuccessful. Cell-type-specific promoters often are leaky, because of either unspecific promoter activity or because of promoter–enhancer trapping events in the case of integrating vectors. Moreover, cell-type-specific promoters are often weak, resulting in low-level transgene expression complicating visualization of reporter genes and functional studies. Furthermore, a microglia-restricted viral envelope is not known to exist. Several recent reports demonstrate the utility of using microRNA (miRNA)-regulated vectors in order to achieve cell-specific transgene expression [10] , [11] , [12] . This system is based on the incorporation of complementary miRNA target sites into the transgene cassette, which leads to degradation of the transgene messenger RNA specifically in cells expressing the miRNA resulting in detargeting of transgene expression. The use of a miRNA-regulated system has several advantages, including the combination of low off-target expression and allow for the use of strong housekeeping promoters. In this study, we demonstrate that miRNA-9 (miR-9)-regulated lentiviral vectors enable robust transgene expression in resident microglia in the rodent brain. Owing to its simplicity and high specificity, this vector will have a broad use for both mechanistic studies as well as novel gene therapy approaches. miR-9-regulated vectors inhibit transgene expression in neural progenitor cells To investigate the expression pattern and activity of miR-9, we generated a lentiviral vector with a housekeeping phosphoglycerate kinase (PGK) promoter driving green fluorescent protein (GFP) expression, coupled with four perfect-match target sequences for miR-9 in the 3′untranslated region (LV.miR-9.T, Fig. 1a ). Thus, when miR-9 is present in the cell, it will bind to the miR-9 target sites and inhibit GFP expression. On the contrary, cells lacking miR-9 will express GFP as the transcript will be processed into protein ( Fig. 1b ). We first used the LV.miR-9.T vector on mouse embryonic stem cells (mES) and mouse neural progenitor cells (mNPC), as it is well established that miR-9 expression is initiated during neural development but absent from embryonic stem cells [13] . When we transduced mES (MOI 50) and mNPC (MOI 10) with LV.miR-9.T or a control GFP lentiviral vector with an identical design but without miR-9 target sites (LV.GFP) ( Fig. 1a ), we found high level of GFP expression in mES ( Fig. 1c ). However, in mNPC we detected little GFP expression when using LV.miR-9.T, corresponding to miR-9 activity in the vast majority of cells, which was in contrast to the high level of GFP expression found when using the LV.GFP control vector ( Fig. 1c ). This demonstrated that LV.miR-9.T was efficiently inhibited in mNPC but not in mES, confirming that miR-9 is active in neural progenitor cells. 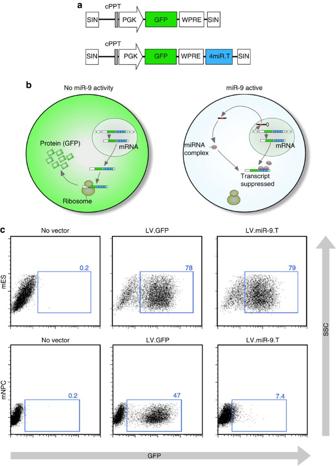Figure 1: Mir-9-regulated vectors are downregulated in NPC. (a) Scheme of the proviral form of LV.GFP and LV.miR-9.T. (b) The vector-encoded transcript is expressed in both miR-9-expressing cell and miR-9-negative cells. In the miR-9-expressing cells, the target containing transcripts are suppressed resulting in loss of GFP expression. (c) Flow cytometry of mES and mNPC transduced with either LV.GFP or LV.miR-9.T demonstrating miR-9 activity only in mNPC. cPPT, central polypurine tract; SIN, self-inactivating; SSC, side scatter. Figure 1: Mir-9-regulated vectors are downregulated in NPC. ( a ) Scheme of the proviral form of LV.GFP and LV.miR-9.T. ( b ) The vector-encoded transcript is expressed in both miR-9-expressing cell and miR-9-negative cells. In the miR-9-expressing cells, the target containing transcripts are suppressed resulting in loss of GFP expression. ( c ) Flow cytometry of mES and mNPC transduced with either LV.GFP or LV.miR-9.T demonstrating miR-9 activity only in mNPC. cPPT, central polypurine tract; SIN, self-inactivating; SSC, side scatter. Full size image Generation of miR-9 sensor transgenic mice We have recently demonstrated that the generation of sensor mice using miR-regulated vectors and lentiviral transgenesis is an efficient and reliable technique to monitor miRNA activity in the brain [14] . This approach has several advantages, including easy colabelling with other immunohistochemical markers, which otherwise is complicated when using alternative miRNA visualizing techniques such as in situ hybridization (ISH) [15] . Also, the reporter system monitors the activity of the miRNA, rather than expression per se , which avoids the influence of potential post-transcriptional regulation, which can be difficult to discriminate when using ISH. To generate sensor transgenic mice, we proceeded to inject high-titre LV.miR-9.T into the periviteline space of fertilized single-cell embryos followed by transfer to surrogate mothers ( Fig. 2a ). We generated four transgenic founders, all carrying multiple copies of the miR-9.T transgene. We intercrossed the different founders and then analysed the F1 generation. In all analysed mice ( n >20) we found reliable GFP expression and there were no differences in the pattern of GFP expression between mice. As a control we used LV.GFP mice, which have been previously characterized [14] . 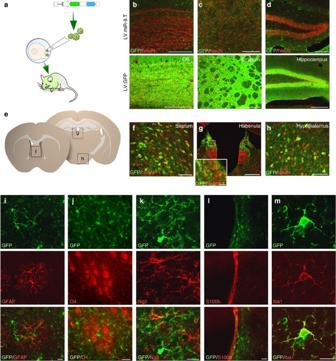Figure 2: Generation and characterization of miR-9.T mice. (a) Illustration of the experimental approach to generate miR-9.T reporter mice using lentiviral transgenesis. Lentiviral vectors were injected into the pervitiline space of fertilized embryos, which were transferred to pseudopregnant mice. (b–d) GFP expression in miR.9.T reporter mice was found exclusively in non-neuronal cells in most brain regions. Control LV.GFP mice displayed GFP expression in all cell types (b–dlower panels). (e–h) GFP-expressing neurons in miR-9.T mice were detected in a few regions close to the midline including the septum, habenula and hypothalamus. (i–l) Confocal analysis demonstrating that astrocytes (GFAP), oligodendrocytes (O4), Ng2-glia (Ng2) and ependymal cells (s100b) express miR-9 (GFP negative), (m) while microglia (Iba1) does not express miR-9 (GFP positive). Scale bars: (b–d) 150 μm; (f) 50 μm; (g) 200 μm; (ginsert) 70 μm; (h) 50 μm; (i–l) 10 μm; (m) 20 μm. Figure 2: Generation and characterization of miR-9.T mice. ( a ) Illustration of the experimental approach to generate miR-9.T reporter mice using lentiviral transgenesis. Lentiviral vectors were injected into the pervitiline space of fertilized embryos, which were transferred to pseudopregnant mice. ( b – d ) GFP expression in miR.9.T reporter mice was found exclusively in non-neuronal cells in most brain regions. Control LV.GFP mice displayed GFP expression in all cell types ( b – d lower panels). ( e – h ) GFP-expressing neurons in miR-9.T mice were detected in a few regions close to the midline including the septum, habenula and hypothalamus. ( i – l ) Confocal analysis demonstrating that astrocytes (GFAP), oligodendrocytes (O4), Ng2-glia (Ng2) and ependymal cells (s100b) express miR-9 (GFP negative), ( m ) while microglia (Iba1) does not express miR-9 (GFP positive). Scale bars: ( b – d ) 150 μm; ( f ) 50 μm; ( g ) 200 μm; ( g insert) 70 μm; ( h ) 50 μm; ( i – l ) 10 μm; ( m ) 20 μm. Full size image miR-9 activity in neurons Analysis of adult brains from miR-9.T mice revealed that most neuronal populations throughout the anterior/posterior axis lacked GFP expression, thus expressing miR-9 (exemplified in Fig. 2b–d by low-magnification images from olfactory bulb, striatum and hippocampus). In most brain regions examined (OB, cortex, striatum, hippocampus, midbrain, cerebellum), we found no GFP-expressing neurons, using immunohistochemistry for GFP and the neuronal marker NeuN ( Fig. 2b–d ). In contrast, LV-GFP control mice displayed high-level GFP expression in NeuN-expressing neurons in these areas ( Fig. 2b–d ). This demonstrated that miR-9 activity is found in the majority of mature neurons in the adult brain. Interestingly, we found GFP expression only in a few discrete neuronal populations that were all aligned close to the midline of the brain in miR-9.T mice. These populations included neurons in the septum, habenula and hypothalamus ( Fig. 2e–h ). NeuN colabelling confirmed the existence of GFP-expressing neurons without miR-9 activity ( Fig. 2f–h ). This demonstrated that miR-9 activity is not an absolute necessity for a neuronal identity. miR-9 activity in glial cells When we examined the non-neuronal cells in the brain we found that astrocytes, oligodendrocytes, NG2-glia and ependymal cells were GFP negative, demonstrating that they displayed miR-9 activity ( Fig. 2i–l ). Instead, the majority of GFP-expressing cells found in the brains of the miR-9.T mice had a morphology typically associated with ramified microglia. Colabelling with the microglia marker, Iba1, confirmed that these cells did not display miR-9 activity ( Fig. 2m ) and we found GFP-expressing microglia throughout the brain. Taken together, this suggests that cells with a neuroectodermal origin, with the exception of a few discrete neuronal populations, display miR-9 activity in the adult mouse brain. However, microglia which constitute the largest population of non-ectodermal cells in the brain do not express miR-9, allowing for easy visualization of these cells in the brain of miR-9.T mice. Targeting resident microglia in vivo With this in mind, we hypothesized that miR-9-regulated vectors may constitute a useful tool to genetically modify specifically resident microglial cells in most brain regions. To this end, we injected LV.miR-9.T vectors or LV.GFP control vectors into the striatum of adult rats ( Fig. 3a ). Four weeks later, rats were killed and the brains processed for histology. 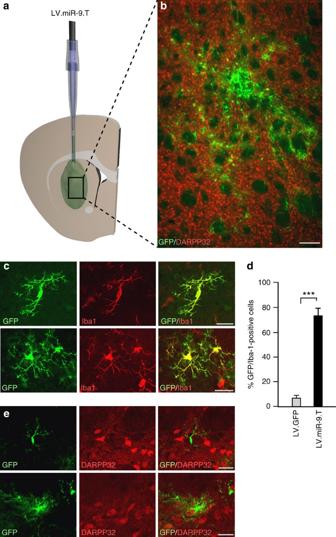Figure 3: Injection of miR-9 into adult rat brain allows visualization of resident microglia. (a) To visualize resident microglia, LV.miR-9-T vectors were injected into rat striatum. Animals were killed 4 weeks later. (b) Large number of GFP-expressing cells with the morphologies of ramified microglia can be detected following injection of LV.miR-9.T. (c) Confocal analysis of two representative ramified microglia colabelling with Iba1. (d) Quantification of the proportion of Iba1/GFP cells in animals injected with LV.miR-9.T (n=5) and a control LV.GFP vector (n=5). (e) GFP-expressing cells do not colabel with the neuronal marker DARPP-32. Scale bars: (b) 100 μm; (c,e) 20 μm. Data are presented as mean±s.e.m. ***P<0.01, Studentst-test. Figure 3: Injection of miR-9 into adult rat brain allows visualization of resident microglia. ( a ) To visualize resident microglia, LV.miR-9-T vectors were injected into rat striatum. Animals were killed 4 weeks later. ( b ) Large number of GFP-expressing cells with the morphologies of ramified microglia can be detected following injection of LV.miR-9.T. ( c ) Confocal analysis of two representative ramified microglia colabelling with Iba1. ( d ) Quantification of the proportion of Iba1/GFP cells in animals injected with LV.miR-9.T ( n =5) and a control LV.GFP vector ( n =5). ( e ) GFP-expressing cells do not colabel with the neuronal marker DARPP-32. Scale bars: ( b ) 100 μm; ( c , e ) 20 μm. Data are presented as mean±s.e.m. *** P <0.01, Students t -test. Full size image The great majority of GFP-expressing cells found after LV.miR-9.T injection displayed typical morphologies of ramified microglia ( Fig. 3b ). We confirmed the microglial identity of the GFP-expressing cells by performing immunohistochemistry for Iba1. Quantifications using confocal microcopy demonstrated that around 75% of GFP-expressing cells were colabelled with Iba1 ( Fig. 3d ). In contrast, we found very few GFP-expressing cells with a neuronal morphology. The proportion of GFP-expressing cells colabelling DARPP-32, a marker for striatal projection neurons was <1% ( Fig. 3e ). We found no GFP-positive cells with an astrocytic morphology. This expression pattern was, as expected, different to what was found after injection of the control LV-GFP vector. In agreement with previous reports [16] , [17] , [18] , we found that when using lentiviral vectors with housekeeping promoters, majority of GFP cells were neurons that colabelled with DARPP-32, while only a small proportion of cells colabelled with microglia markers ( Fig. 3d ). In summary, this experiment demonstrated that miR-9 target sites are capable of repressing transgene expression in non-microglial cell types following vector injection into the adult rat brain, allowing high-level transgene expression specifically in resident microglia. miR-9 vectors allow monitoring of activated microglia Thereafter, the LV.miR-9.T vector was used to visualize and isolate activated resident microglia after an excitotoxic insult. This type of experiment has been difficult to achieve using previous genetic modification techniques, as it has been problematic to distinguish resident microglia from the infiltrating monocytes/macrophages that enter the brain following several pathological stimuli. To visualize the response of endogenous microglia to a toxic lesion, we injected LV.miR-9.T vectors into the striatum of adult rats. A parenchymal vector injection will result in genetic modification only of the resident microglia, while circulating monocyte cells will not be transduced with the vector. Thus, all GFP-expressing microglia that we detect will be derived from the resident population. Three weeks after vector injection, the rats received an excitotoxic ibotenic acid lesion ( Fig. 4a ). The rats were then killed 1 week after lesion. We chose this lesion paradigm as it leads to a strong glial response, including microglia activation [19] , [20] . 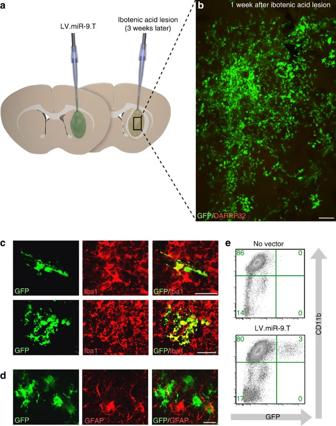Figure 4: Visualization of activated microglia. (a) LV.miR-9.T vectors were injected into rat striatum. Three weeks later, rats received an excitotoxic ibotenic acid lesion in the striatum. Animals were killed 1 week later. (b) Large numbers of GFP-expressing cells with the morphologies of activated microglia were found after injection of LV.miR-9.T followed by an excitotoxic lesion. Note the lack of DARPP-32 staining due to neuronal loss following lesion. (c) Confocal analysis of typical activated resident microglia colabelling with Iba1. (d) GFP-stained cells do not overlap with the astrocyte marker GFAP. (e) FACS plot of GFP/CD11b-expressing cells from isolated from freshly dissected lesioned striatum. GFP-expressing cells corresponded to on average 3.4±1.2% (n=4) of the CD11b cells present in the brain. Scale bars: (b) 100 μm; (c,d) 20 μm. Figure 4: Visualization of activated microglia. ( a ) LV.miR-9.T vectors were injected into rat striatum. Three weeks later, rats received an excitotoxic ibotenic acid lesion in the striatum. Animals were killed 1 week later. ( b ) Large numbers of GFP-expressing cells with the morphologies of activated microglia were found after injection of LV.miR-9.T followed by an excitotoxic lesion. Note the lack of DARPP-32 staining due to neuronal loss following lesion. ( c ) Confocal analysis of typical activated resident microglia colabelling with Iba1. ( d ) GFP-stained cells do not overlap with the astrocyte marker GFAP. ( e ) FACS plot of GFP/CD11b-expressing cells from isolated from freshly dissected lesioned striatum. GFP-expressing cells corresponded to on average 3.4±1.2% ( n =4) of the CD11b cells present in the brain. Scale bars: ( b ) 100 μm; ( c , d ) 20 μm. Full size image One set of rats was used for histology. In the lesioned brains injected with LV.miR-9.T, we detected numerous GFP-expressing cells with the typical morphology of activated microglia ( Fig. 4b ). These GFP+ cells also colabelled with Iba1 ( Fig. 4c ). It is worth noting that there was an extensive upregulation of Iba1 immunoreactivity to which infiltrating monocytes/macrophages are likely to contribute. We detected very limited GFP expression in glial fibrillary acidic protein (GFAP)-expressing astrocytes, a cell type which is also activated following an excitotoxic lesion ( Fig. 4d ) [21] . In the second set of animals, lesioned striatal tissue was freshly dissected, prepared into a single-cell suspension and analysed using flow cytometry to determine the percentage of GFP-expressing cells in the myeloid (CD11b) cell fraction in brains where there is infiltration from the circulating myeloid population. We found that with the injection protocol used, GFP-expressing cells corresponded to on average 3.4±1.2% ( n =4) of the CD11b cells present in the brain, showing that with a single-site vector injection we reach a substantial fraction of the resident microglia in the rat striatum and distinguish it from the circulation pool of myeloid cells ( Fig. 4e ). Using cell sorting we were able to obtain on average about 600 cells per animal using this procedure, which is a sufficient number of cells for most downstream molecular approaches such as quantitative real-time PCR, microarray or RNA-seq. It is also worth noting that almost all GFP-expressing cells (>99%, n =4) also expressed CD11b, further demonstrating the specificity of the LV.miR-9.T-vector. Thus, this experiment demonstrated that LV.miR-9.T vectors could be used both to monitor and isolate the activated resident microglia following a lesion and hereby efficiently separate the resident population of microglia from cells infiltrating from the blood. In this study we used a miR-9-regulated lentiviral vector to target resident microglia after injection into the adult rodent brain. The use of miR-9 target sites ensures that GFP expression is found only in cells with a non-ectodermal origin including microglia. The use of an intra-parenchymal vector injection ensures that only the resident microglia population is genetically modified. Thus, combining a parenchymal injection of a viral vector and a cell-type-specific expression allows visualization and genetic modification of resident microglia without affecting circulating monocytes/macrophages. A potential drawback with this approach is its invasive nature, which may in itself cause microglia activation. However, there are several reports demonstrating that injection of lentiviral vectors into the brain is associated with minimal microglia activation (see, for example, refs 16 , 22 ). This was also evident in the current study as the majority of the GFP-expressing cells were non-activated ramified microglia ( Fig. 3b ). Taken this into account, the microglia-specific miR-9-regulated vector offers rapid and straightforward experimental approaches in combination with high specificity and should be a valuable tool to study the role of resident microglia in the healthy and diseased brain. Key to our approach was the generation of a miR-9 sensor transgenic mouse that provided a detailed expression map of miR-9 activity in the brain. Although this approach does not take into account the absolute expression level or the stability of the miRNA, [23] the use of sensor mice has several advantages over LNA fluorescent ISH, which is the most commonly used method to analyse the expression pattern of individual miRNA in the brain. In particular, the use of a GFP reporter is suitable for colabelling with other markers, here highlighted by the identification of Iba1-expressing microglia as miR-9 negative. The expression pattern of miR-9 in mouse brain was previously poorly characterized and the finding that microglia does not express miR-9 opened up for the possibility to use miR-9 target sites as a useful technique to target transgene expression to microglia. In recent years, vectors encompassing miR target sites have become an efficient tool to target transgene expression to certain cell populations. The main advantage of miR-regulated vectors is the highly robust downregulation of transgene expression, which occurs when the regulating miRNA is present in the cell. This advantage is combined with a strong housekeeping promoter in the vector. Our study further supports the concept of using miR-regulated vectors to achieve cell-type-specific transgene expression, for either experimental studies or gene therapy purposes. Another advantage of miR-regulated vectors is that they often can be directly transferred between species because of the large degree of conservation of mature miRNA sequences. In our study this is demonstrated by the use of miR-9 vectors in both mice and rats. However, it should be noted that it is unclear how conserved the expression pattern of different brain enriched miRNAs is between rodents and humans, and it remains to be tested whether miR-9-regulated vectors can be used also to target human microglia. Our study also glances into the functional role of miR-9 in the adult mouse brain. miR-9 has previously been implicated in migration, differentiation and maturation of neural progenitors by regulating multiple transcription factors [13] , [24] . Furthermore, miR-9 has been demonstrated to act in concert with miR-124 to establish neuronal identity [25] . In fact, coexpression of miR-9 and miR-124 is sufficient to induce functional neuronal cells directly from fibroblasts [26] . However, our results suggest that miR-9 and miR-124 do not have exactly overlapping functions. While miR-124 is exclusively found in neurons or cells destined to become neurons [14] , miR-9 is expressed in all neuroectodermal lineages including neurons, astrocytes, ependymal cells and oligodendrocytes. It is also interesting to note that miR-9 is absent from a small number of neuronal nuclei in the adult mouse brain. This suggests that some neuronal populations have unique transcriptional profiles that are not under the influence of miR-9 regulation. Investigations of the functional consequence of this phenomenon will be very interesting. In summary, we have monitored the activity of miR-9 in the adult rodent brain and demonstrate the ability of miR-9-regulated vectors to specifically target transgene expression to microglia. These vectors have great potential for the studies of microglial function in both the healthy and diseased brain. Viral vectors The lentiviral vectors used in this study were third-generation self-inactivating vectors. miRNA target sequences were cloned into the 3′-untranslated region of the transgene expression cassette. A detailed description on how to generate lenviral vectors with miRNA target sequences have been described elsewhere [10] . The target sequence for miR-9 is 5′-TCATACAGCTAGATAACCAAAG-3′ ( www.mirbase.org ). The four target sites were cloned immediately downstream the woodchuck hepatitis virus post-transcriptional response element (WPRE) of a third-generation lentiviral vector, expressing GFP from the PGK promoter derived from the phosphoglycerol kinase housekeeping gene. This promoter results in robust, ubiquitous moderate level transgene expression, with very low tendency to transgene silencing/variegation. Lentiviral vectors were produced as previously described [27] . These vectors were titrated using flow cytometry and quantitative PCR analysis as previously described [28] . The titres of the vectors in this study were in the range of: 5 × 10 8 –1 × 10 9 TU per ml. Cell culture Mouse NPC cells were derived from E14 mouse ES cells and cultured as previously described [29] . E14 mouse ES cells were maintained as previously described with minor modifications [30] . Briefly, cells were expanded in Dulbecco’s Modified Eagles Medium (DMEM, Gibco) supplemented with 10% fetal calf serum (BioSera), non-essential amino acids (Gibco), sodium pyruvate (Gibco) glutamine (Sigma Aldrich), penicillin/streptomycin (Sigma Aldrich) and leukaemia inhibitory factor on gelatin-coated culture flasks (Nunc). Every second day the cells were passaged using trypsin and plated at a density of 4 × 10 4 cells cm −2 . Animals All animal-related procedures were approved by and conducted in accordance with the committee for use of laboratory animals at Lund University and EPFL. Lentiviral trangenesis was performed as previously described [31] . Offspring were genotyped and number of integrated transgenes was estimated using quantitative real-time PCR. Primers: WPRE fw: 5′-GGCACTGACAATTCCGTGGT-3′, rev: 5′-AGGGACGTAGCAGAAGGACG-3′. Probe WPRE 5′-ACGTCCTTTCCATGGCTGCTCGC-3′. Titine fw: 5′-AAAACGAGCAGTGACGTGAGC-3′, rev: 5′-TTCAGTCATGCTGCTAGCGC-3′. Probe Titine 5′-TCGACGGAAGCGTCTCGTCTCAGTC-3′. The data were quantified using the ΔΔCt-method. The transgene data (WPRE primer) was normalized with the Titine data to give the number of transgenes in the genome of each animal. For vector injections into adult rats ( n =10), female Sprague–Dawley rats (Charles River) weighing 200–250 g were used. One microlitre of lentiviral vector (LV.PGK.GFP or LV.PGK.GFP.miR.9.T) was injected bilaterally into the rat striatum. A thin glass capillary was attached to a Hamilton syringe to diminish the artifact damage resulting from stereotaxic injection. The stereotaxic injection coordinates were TB=0, AP +1.2, ML ±2.5 and DV −4.5 mm from bregma [32] . A total of 14 μg (1.4 μl, 0.4–0.5 μl per site) of ibotenic acid (10 μg ml −1 in 0.1 M of phosphate buffer, supplier Sigma) was injected unilaterally into rat striatum (right hemisphere) in three different sites. The stereotaxic injection coordinates were: TB −2.3 mm, AP +1.5 mm, ML −3 mm, DV 1–5.6 mm, and AP +1.2 mm, ML −3 mm and DV −4/−5.5 mm from the bregma [32] . Immunofluorescence Mice and rats were transcardially perfused with 4% paraformaldehyde (Sigma), the brains post-fixed for 2 h and transferred to PBS with 25% sucrose. Brains were coronally sectioned on a microtome (35 μm) and put in phosphate-buffered saline with potassium (KPBS). The procedure for immunohistochemistry has been published in detail elsewhere [12] , [33] . Primary antibodies were diluted as follows: chicken anti-GFP 1:1,000 (Abcam), rabbit anti-GFAP 1:1,000 (DAKO), mouse anti-NeuN 1:1,000 (Millipore), rabbit anti-Iba1 1:1,000 (WAKO), mouse anti-S100b 1:500 (Sigma), mouse anti-O4 1:100 (Millipore), rabbit anti-Ng2 1:200 (Millipore), rabbit-anti-DARPP-32 1:1,000 (Chemicon). The dilution factor of the secondary antibodies was 1:500 (Molecular Probes) or 1:200 (Jackson Laboratories). Flow cytometry Microglia were isolated as previously described with minor modifications [34] . Rats were decapitated, brains were rapidly removed and placed in Leibovitz-15 media. The entire lesioned striatum was micro-dissected under a dissection microscope in L15 media. The tissue was diced and resuspended in a 37-°C papain, neutral protease (dispase II) and DNAse solution, and incubated for 30 min at 37 °C. Tissue was then tritrated, and excess DMEM/F12 with glutamine (500 μl per 50 ml) and 10% fetal bovine serum (media) was added. Next, cells were washed by centrifugation, resuspended in media and strained through a 40-μm strainer. Cells were recentrifuged and resuspended in 4 ml 37% percoll in media. Four millilitres of 70% percoll was slowly underlaid and 30% percoll added on top followed by an additional 2 ml of media. A gradient was run for 40 min, 200 × g , 18 °C. The thick viscous layer of debris formed was removed and the halo-like ring of microglia formed between the 70 and 37% gradients was collected and washed by centrifugation in media. Cells were then resuspended in fluorescence-activated cell sorting (FACS) block buffer (0.1% fetal bovine serum in PBS) with allophycocyanin (APC)-conjugated mouse anti-rat CD11b (1:100; Invitrogen) for 30 min at 4 °C. Cells were then washed by centrifugation at 4 °C and resuspended in 400 μl FACS buffer (1% bovine serum albumin (BSA) in PBS) ready for FACS analysis using a BD FACS Aria III (BD Biosciences). Two minutes before sorting, 2 μl propidium iodide (Sigma Aldrich, Germany) was added to the sample for the identification of dead cells. Quantification To quantify the proportion of microglial cells transduced by LV.GFP and LV.miR-9.T, GFP-expressing cells were analysed throughout the whole transduced area. The needle tract and adjacent areas were excluded to avoid interference by artifacts caused by the localized inflammation resulting from stereotaxic injection. Images (six) were captured using confocal microscopy from each section with GFP-expressing cells. GFP-positive cells colabelled with Iba1 were considered microglia. An unpaired T -test was performed to test for statistical significance. Data are presented as mean±s.e.m. How to cite this article: Åkerblom, M. et al . Visualization and genetic modification of resident brain microglia using lentiviral vectors regulated by microRNA-9. Nat. Commun. 4:1770 doi: 10.1038/ncomms2801 (2013).